Stress-induced inactivation of theStaphylococcus aureuspurine biosynthesis repressor leads to hypervirulence Staphylococcus aureus is a significant cause of human infection. Here, we demonstrate that mutations in the transcriptional repressor of purine biosynthesis, purR , enhance the pathogenic potential of S. aureus . Indeed, systemic infection with purR mutants causes accelerated mortality in mice, which is due to aberrant up-regulation of fibronectin binding proteins (FnBPs). Remarkably, purR mutations can arise upon exposure of S. aureus to stress, such as an intact immune system. In humans, naturally occurring anti-FnBP antibodies exist that, while not protective against recurrent S. aureus infection, ostensibly protect against hypervirulent S. aureus infections. Vaccination studies support this notion, where anti-Fnb antibodies in mice protect against purR hypervirulence. These findings provide a novel link between purine metabolism and virulence in S. aureus . In humans, Staphylococcus aureus may exist as a commensal bacterium or as a pathogen. Data from the United States Centers for Disease Control and Prevention show that approximately one-third of the US population is colonized with S. aureus [1] , and colonization with S. aureus is associated with increased risk of subsequent infection [2] . Infections caused by S. aureus range in severity from relatively minor skin and soft tissue infections through to invasive diseases such as pneumonia, infective endocarditis and osteomyelitis [3] . Strikingly, the magnitude of morbidity and mortality caused by S. aureus is highlighted by reports that, in the US, invasive infections by this bacterium cause more deaths than HIV [4] . That S. aureus can infect virtually any organ or tissue in the body is a reflection of its vast repertoire of virulence factors that contribute to bacterial pathogenesis through mechanisms involving tissue adherence [5] , [6] , cellular intoxication [7] , [8] , [9] , and immune modulation and deception [10] , [11] . Virulence factor expression in S. aureus is complex and coordinately regulated by multiple transcription factors, regulatory RNAs, two-component sensing systems and quorum-sensing [12] , [13] , [14] . Despite a wealth of knowledge on virulence regulation in S. aureus , there are still outstanding questions to be resolved, as novel mechanisms of virulence regulation are still being discovered, especially with regard to environmental or metabolic cues to which S. aureus responds [15] . Exposure to elevated temperatures, for example 42 °C, a temperature frequently used to cure S. aureus of recombinant plasmids during mutagenesis procedures, can select for mutations in the S. aureus genome. Mutations in the global two-component regulator SaeRS have previously been isolated following mutagenesis [16] , and mutations in the sae regulatory system show drastically reduced toxin production and have attenuated virulence [17] , [18] , [19] , [20] . Screening for unintended sae mutations is straight forward, as the mutants are easily identified as having reduced haemolytic activity on blood agar plates. Little is known, however, about other unintended secondary mutations that may be selected for in response to stress, especially those that may impact on the virulence potential of S. aureus . In this study, we identify mutations that occur in the S. aureus purR gene in response to stress, including growth at elevated temperatures (i.e. 42 °C). The function of purR in S. aureus has not been characterized, but the gene is homologous to those that encode the purine biosynthesis repressors in Bacillus subtilis and Escherichia coli ; we show here that mutations in purR do indeed result in upregulation of purine biosynthetic genes in S. aureus . However, we further demonstrate that purR mutations have a heretofore undescribed role in regulating expression of S. aureus fibronectin binding proteins and, thus, play a role in the interaction of S. aureus with fibronectin. In the absence of anti-FnbA/B antibodies, purR mutants clump vigorously in serum in a fibronectin-dependent manner. Importantly, purR mutants, also through FnbA/B-dependent mechanisms, are hypervirulent in a systemic model of infection in mice, and vaccination of mice against FnbA/B can diminish hypervirulence and ameliorate animal mortality. We suggest that, in S. aureus , PurR is critical to limit the expression of fnb genes, known to be maximally expressed at low cell density, in order to promote colonization, yet prevent cell clumping in the vasculature. S. aureus purR mutants vigorously clump during growth in serum In our laboratory, we generate deletion mutations in iron-regulated genes and test mutants for growth in chemically defined media (e.g. RPMI-1640) containing 10% v/v horse serum (HS) to induce iron starvation. Over time, we noted that a number of mutants, in the USA300 genetic background, would clump vigorously when grown in the presence of HS, a trait not observed for WT USA300. The hallmark of this phenotype was that, during growth, visibly large clumps would appear in the culture and, when the culture tube was allowed to sit without shaking, the clumped material would settle to the bottom of the tube within minutes. This response was independent of iron starvation as robust clumping occurred when the bacteria were grown in tryptic soy broth, an iron replete medium, containing 10% v/v HS (TSB-S). To investigate this phenotype further, we performed whole genome sequencing on one of these clumping mutants and identified a non-synonymous single nucleotide polymorphism (SNP) in the purR gene causing a Q52P mutation ( purR Q52P ). The purR gene is homologous to those encoding the purine biosynthesis repressors in E. coli and B. subtilis but, to date, has not been studied in S. aureus . We independently discovered a second clumping mutant while generating a completely separate markerless deletion in the USA300 genome. We PCR-amplified the purR gene and discovered it carried a deletion of a guanine at position 682 of the gene, causing a frameshift in the protein after V229. To confirm that loss of purR indeed correlated with the hyper-clumping phenotype, we mobilized the purR ::ΦNΣ mutation from the Nebraska transposon mutant library [21] into our laboratory USA300 strain (hereafter referred to as purR ::ΦNΣ). The purR ::ΦNΣ strain demonstrated similar clumping to the SNP-containing strain and the phenotype could be fully complemented by providing purR in trans on a multi-copy plasmid (referred to as p purR ) (Fig. 1a ). Given that cultures containing clumped bacteria, when allowed to sit without shaking, rapidly clarify due to sedimentation of the cells in culture tubes, we developed an assay to quantitate relative clumping by measuring the culture optical density (see the Methods section). This analysis detected a significant decrease in OD 600 values for both WT USA300 and purR ::ΦNΣ in TSB-S, when compared to TSB alone. However, bacterial sedimentation (i.e. clumping) was greatly enhanced for purR ::ΦNΣ in serum as compared to WT USA300 (Fig. 1b ). Furthermore, these measurements confirmed that provision of purR in trans completely reversed the clumping phenotype (Fig. 1b ). Fig. 1 Disruption of purR causes cell clumping of S. aureus USA300. In a , representative images of USA300, USA300 purR ::ΦNΣ or the complemented purR ::ΦNΣ mutant in culture tubes following growth in TSB with 10% (v/v) horse serum (TSB-S) for 3.5 h from a starting OD 600 equivalent of 0.03. In b , graphical representation of the relative sedimentation of bacterial aggregates in cultures as grown in a , reflected by the OD 600 values of the centre of liquid cultures after sitting without shaking for 5 min following shaking at 37 °C for 3.5 h. Data are mean ± SEM of four independent experiments. *** p- value < 0.001, based on a one-way analysis of variance (ANOVA) with a Bonferroni post-test. In c , the representative micrographs show bacterial cell clusters that arise during growth in TSB or TSB-S. White boxes define the region of interest that is depicted in the insets. Scale bars  = 40 µm. In d , transmission electron micrographs are shown for S. aureus USA300 and the USA300 purR ::ΦNΣ strain grown in the presence (TSB-S) or absence (TSB) of horse serum. The representative images depict cells at ×11,000 magnification. Scale bars  = 1 µm. Source data are provided as a Source Data file Full size image To study the hyper-clumping phenotype further, we used brightfield microscopy to examine the cells grown in TSB or TSB-S. WT USA300 and the complemented purR ::ΦNΣ mutant grown in TSB formed only small ‘grape-like’ clusters of 2–4 cells, as expected for S. aureus . In contrast, purR ::ΦNΣ formed aggregates comprised of greater numbers of cells, including some noticeably larger clusters that were not observed for WT bacteria (Fig. 1c , top panels). Consistent with what is known of the interaction of S. aureus with serum proteins [22] , [23] , USA300 and the purR ::ΦNΣ complemented strains, grown in TSB-S as compared to TSB alone, formed larger cell clusters due to aggregation of the bacteria through binding of serum proteins (Fig. 1c , bottom panels). In contrast, bacterial aggregation was greatly exaggerated for purR ::ΦNΣ, where aggregated masses of bacteria took up the majority of the field of view (Fig. 1c , bottom panel), undoubtedly related to the macroscopic sedimentation observed in liquid cultures. To assess whether cell clumping could be caused by cell division defects in the purR ::ΦNΣ background, we performed transmission electron microscopy of WT or purR ::ΦNΣ mutant cells grown in TSB or TSB-S. For both strains, irrespective of culture conditions, division septa were visible and the apparent cell morphology did not differ, indicating cell division defects were not present in purR ::ΦNΣ (Fig. 1d ). We therefore next hypothesized that the robust aggregation of purR bacteria was mediated by specific bacterial factors. 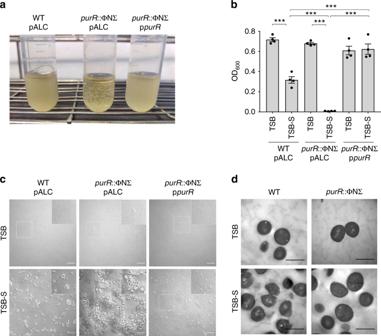Fig. 1 Disruption ofpurRcauses cell clumping ofS. aureusUSA300. Ina, representative images of USA300, USA300purR::ΦNΣ or the complementedpurR::ΦNΣ mutant in culture tubes following growth in TSB with 10% (v/v) horse serum (TSB-S) for 3.5 h from a starting OD600equivalent of 0.03. Inb, graphical representation of the relative sedimentation of bacterial aggregates in cultures as grown ina, reflected by the OD600values of the centre of liquid cultures after sitting without shaking for 5 min following shaking at 37 °C for 3.5 h. Data are mean ± SEM of four independent experiments. ***p-value < 0.001, based on a one-way analysis of variance (ANOVA) with a Bonferroni post-test. Inc, the representative micrographs show bacterial cell clusters that arise during growth in TSB or TSB-S. White boxes define the region of interest that is depicted in the insets. Scale bars  = 40 µm. Ind, transmission electron micrographs are shown forS. aureusUSA300 and the USA300purR::ΦNΣ strain grown in the presence (TSB-S) or absence (TSB) of horse serum. The representative images depict cells at ×11,000 magnification. Scale bars  = 1 µm. Source data are provided as aSource Datafile Interestingly, no discernible differences in protein profiles or growth were observed between WT and purR ::ΦNΣ bacteria at various growth phases (Supplementary Figure 1a, b, c ). RNAseq on mid-exponential (OD 600 = 1.0) phase cultures grown in TSB showed that genes of the purine biosynthesis pathway were elevated in the purR ::ΦNΣ strain, as compared to the WT, however, few other differences could be detected between the two genotypes (Supplementary Table 1 ). RT-PCR was performed on a select number of genes and the data agreed with the RNAseq data, where purE , the first gene in the purEKCSQLFMNHD purine biosynthetic operon, demonstrated the greatest transcriptional increase (Supplementary Figure 1d ). Altogether, these data demonstrate that purR regulates the purine biosynthesis pathway of S. aureus and inactivation of purR leads to exaggerated serum-dependent cell clustering. However, these analyses failed to identify an obvious effector responsible for the clumping phenotype. Serum clumping requires fibronectin binding proteins We next analysed whether the purR phenotype was conserved across different S. aureus backgrounds. To this end, we transduced the purR ::ΦNΣ mutation into S. aureus strains RN6390, SH1000, MN8 and Newman and complemented each mutant. 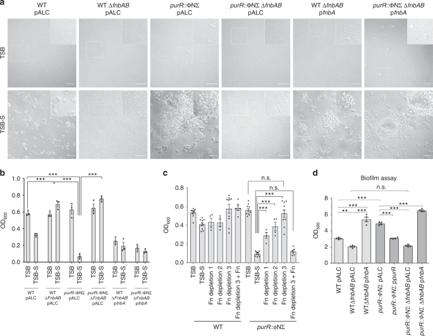Fig. 2 ThepurR-dependent clumping phenotype requires fibronectin binding proteins and host fibronectin. Ina, cultures were grown in TSB or TSB-S for 3.5 h and then imaged on a wide field microscope at ×40 magnification. White boxes define the region of interest that is depicted in the insets. Scale bars = 40 µm. Representative images are shown. Inb, cultures were grown as inaand OD600was measured as described in the legend to Fig.1and in the Methods section. Data shown are mean ± SEM of four independent experiments. ***p-value < 0.001, based on a one-way ANOVA with a Bonferroni post-test. Inc, WT and thepurR::ΦNΣ mutant were grown in TSB, TSB-S, TSB containing 10% v/v of various levels of Fn-depleted horse serum or Fn-depleted horse serum with the addition of eluted fibronectin (Fn depletion 3+Fn). Measurement of OD600of cultures to evaluate clumping was performed as described above. Data shown are mean ± SEM of five independent experiments and two different Fn purifications. ***p-value < 0.001, based on a one-way ANOVA with a Bonferroni post-test. Ind, biofilm forming ability of indicated strains was measured after growth in TSB in a standard 96-well plate biofilm assay (see the Methods section). Data shown are mean ± SEM of four experiments. **p-value < 0.01, ***p-value < 0.001, based on a one-way ANOVA with a Bonferroni post-test. Source data are provided as aSource Datafile Similar to USA300, growth of the RN6390, SH1000 and MN8 purR mutants in TSB-S demonstrated vigorous cell clumping and, for each strain, provision of purR in trans complemented the phenotype (Supplementary Figure 2a, b, c ). In contrast, Newman purR ::ΦNΣ failed to hyper-aggregate in the presence of HS and was indistinguishable from WT Newman when grown in either TSB or TSB-S (Supplementary Figure 2d ). Of note, strain Newman expresses mutated fibronectin binding proteins (FnBPs; FnbA and FnbB) that, unlike in other S. aureus strains, are not cell wall anchored [24] , leading us to hypothesize that cell wall anchored FnbA/B may be required for hyper-clumping. To directly test the involvement of the FnBPs in purR -dependent clumping, we engineered, in WT and purR ::ΦNΣ USA300 bacteria, markerless deletions of the tandemly-duplicated fnbA and fnbB genes. Growth of the resulting purR ::ΦNΣ fnbA/B mutants in TSB and TSB-S did not differ from that of WT USA300 and, notably, serum-dependent hyper-clumping did not occur (Fig. 2a, b ). Indeed, the USA300Δ fnbAB construct exhibited less serum-dependent clumping than WT, demonstrating the importance of these proteins in normal interactions of S. aureus with serum components (Fig. 2a ). Of note, complementation of the Δ fnbAB mutants with fnbA on an overexpression plasmid resulted in exaggerated clumping during growth in TSB without serum (Fig. 2a, b ), likely due to the increased number of homophilic interactions between FnbA molecules, which have previously been reported to contribute to bacterial aggregation [25] . Overall, these data show that hyper-clumping due to purR inactivation occurs in several S. aureus strains and requires cell wall-anchoring of FnBPs. Fig. 2 The purR -dependent clumping phenotype requires fibronectin binding proteins and host fibronectin. In a , cultures were grown in TSB or TSB-S for 3.5 h and then imaged on a wide field microscope at ×40 magnification. White boxes define the region of interest that is depicted in the insets. Scale bars = 40 µm. Representative images are shown. In b , cultures were grown as in a and OD 600 was measured as described in the legend to Fig. 1 and in the Methods section. Data shown are mean ± SEM of four independent experiments. *** p -value < 0.001, based on a one-way ANOVA with a Bonferroni post-test. In c , WT and the purR ::ΦNΣ mutant were grown in TSB, TSB-S, TSB containing 10% v/v of various levels of Fn-depleted horse serum or Fn-depleted horse serum with the addition of eluted fibronectin (Fn depletion 3+Fn). Measurement of OD 600 of cultures to evaluate clumping was performed as described above. Data shown are mean ± SEM of five independent experiments and two different Fn purifications. *** p -value < 0.001, based on a one-way ANOVA with a Bonferroni post-test. In d , biofilm forming ability of indicated strains was measured after growth in TSB in a standard 96-well plate biofilm assay (see the Methods section). Data shown are mean ± SEM of four experiments. ** p -value < 0.01, *** p- value < 0.001, based on a one-way ANOVA with a Bonferroni post-test. Source data are provided as a Source Data file Full size image Serum clumping by purR mutants requires fibronectin The multifunctional S. aureus FnBPs bind to fibrinogen, fibronectin and elastin [5] . To determine which serum component was involved in the clumping phenotype, we allowed purR ::ΦNΣ bacteria to grow in TSB-S and form clumps. We isolated the clumped material and used mass spectrometry to identify enriched serum proteins that copurified with the bacteria (see the Methods section). These analyses revealed only one protein, fibronectin (Fn) from Equus ferus przewalskii (Mongolian wild horse) was significantly enriched in purR ::ΦNΣ derived samples. 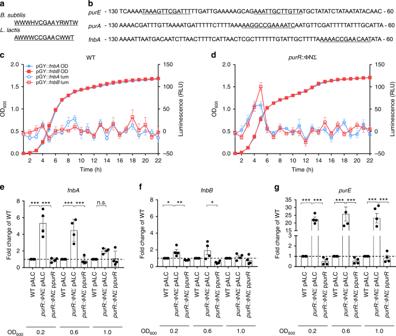Fig. 3 purRmutations lead to transcriptional upregulation of the purine biosynthesis operon andfnbAB.aConsensus PurBox sequence forB. subtilisandL. lactis(data adapted from refs.26,27).bPromoter sequences ofpurE,purAandfnbA, with putative PurBox sequences underlined. WT (c) orpurR::ΦNΣ mutant (d) containing a luciferase construct with the promoter sequence offnbAorfnbB(see the Methods section) were grown in TSB and OD600and luminescence monitored. Data shown are mean ± SEM of three experiments. Ine,fandg, indicated strains were grown to OD600of 0.2, 0.6 or 1.0, total RNA was extracted and RT-PCR analysis performed for relative abundance offnbA(e),fnbB(f) andpurE(g) transcripts. All data were normalized to levels ofrpoBand expressed as fold change using WT pALC (empty plasmid) as comparator at each OD600value. Data shown are mean ± SEM of four independent experiments. *p-value < 0.05, **p-value < 0.01, ***p-value < 0.001, based on a one-way ANOVA with a Bonferroni post-test. Source data are provided as aSource Datafile To confirm the involvement of Fn in purR -dependent hyper-clumping, soluble Fn was removed from horse serum by serial passage over a gelatin sepharose column (Supplementary Figure 3 ). When the Fn-depleted serum was used in clumping assays, we observed a decrease in the hyper-clumping phenotype of the purR ::ΦNΣ mutant (Fig. 2c ). Reconstitution of the Fn-depleted serum with the purified horse Fn restored purR -dependent clumping to normal levels (Fig. 2c ). Together these data demonstrate the purR- dependent clumping in serum requires S. aureus FnBPs and host Fn. S. aureus purR mutants demonstrate enhanced biofilm formation The clustering of purR ::ΦNΣ cells in TSB, coupled with the dependency of the aggregation phenotype on FnBPs, lead us to hypothesise that purR ::ΦNΣ bacteria were better able to initiate biofilm formation. In agreement, purR ::ΦNΣ bacteria formed increased biofilm as compared to WT USA300 (Fig. 2d ), and this phenotype could be eliminated by the deletion of fnbAB in the purR ::ΦNΣ background (Fig. 2d ). Moreover, deletion of fnbAB genes eliminated any differences between WT and purR ::ΦNΣ cells and diminished biofilm formation. Conversely, overexpression of fnbA from a plasmid enhanced biofilm formation, irrespective of purR . PurR represses transcription of the purE operon and fnbAB How inactivation of purR is connected to FnBP function and/or expression was not understood, since our RNAseq analysis failed to detect changes in either fnbA or fnbB transcript levels at culture densities of OD 600 of 1.0. Studies in B. subtilis and Lactococcus lactis have identified conserved sequence motifs in promoter regions, named PurBoxes, where PurR binds. Single or double PurBoxes can be present, and double PurBoxes are often palindromic, but all contain a central conserved CGAA motif [26] , [27] (Fig. 3a ). Analysis of the S. aureus genome identified sequences similar to those in B. subtilis and L. lactis upstream of the purE and purA genes in S. aureus USA300 (Fig. 3b ) and, not surprisingly, these genes are upregulated in the purR ::ΦNΣ strain (see Supplementary Table 1 ). Remarkably, a similar putative PurR-binding sequence was also present upstream the fnbA and fnbB genes (Fig. 3b ). To determine whether transcription of fnbA and fnbB is influenced by PurR we generated plasmids carrying the fnbA and fnbB promoters fused to a promoterless lux -gene construct and monitored bioluminescence in WT and purR ::ΦNΣ bacteria. Bioluminescence could not be detected above background levels in WT cells, presumably due to low levels of transcription from the fnb A/B promoters (Fig. 3c ). In contrast, bioluminescence was detected for both the fnbA and fnbB promoter constructs in the purR ::ΦNΣ mutant, where luminescence peaked at a culture density of OD 600 0.5–0.6 (Fig. 3d ). Accordingly, we investigated transcript levels of fnbA and fnbB at early growth phases. Relative to WT, fnbA transcripts were elevated in the purR ::ΦNΣ mutant, at culture densities as low as OD 600 of 0.2 (Fig. 3e ), and steadily decreased as the culture density increased. Consistent with our RNAseq analysis, no significant differences in fnbA transcripts were present between the WT and the purR ::ΦNΣ mutant at an OD 600 of 1.0. Of note, fnbB transcripts were only elevated in the purR ::ΦNΣ mutant at OD 600 of 0.2 (Fig. 3f ). Consistent with de-repression due to the absence of its regulator/repressor, and concordant with our previous data, purE transcripts were upregulated at all time points tested (Fig. 3g ). Fig. 3 purR mutations lead to transcriptional upregulation of the purine biosynthesis operon and fnbAB . a Consensus PurBox sequence for B. subtilis and L. lactis (data adapted from refs. [26] , [27] ). b Promoter sequences of purE , purA and fnbA , with putative PurBox sequences underlined. WT ( c ) or purR ::ΦNΣ mutant ( d ) containing a luciferase construct with the promoter sequence of fnbA or fnbB (see the Methods section) were grown in TSB and OD 600 and luminescence monitored. Data shown are mean ± SEM of three experiments. In e , f and g , indicated strains were grown to OD 600 of 0.2, 0.6 or 1.0, total RNA was extracted and RT-PCR analysis performed for relative abundance of fnbA ( e ), fnbB ( f ) and purE ( g ) transcripts. All data were normalized to levels of rpoB and expressed as fold change using WT pALC (empty plasmid) as comparator at each OD 600 value. Data shown are mean ± SEM of four independent experiments. * p -value < 0.05, ** p -value < 0.01, *** p -value < 0.001, based on a one-way ANOVA with a Bonferroni post-test. Source data are provided as a Source Data file Full size image S. aureus purR mutants are hypervirulent Given the strong Fn-binding phenotype associated with a S. aureus purR mutant, we evaluated the virulence potential of the mutant. Mice were infected via the tail vein with WT USA300, the purR ::ΦNΣ mutant, and the purR ::ΦNΣ mutant complemented with p purR at a dose of ~1 × 10 7 CFU. Remarkably, 100% of the mice infected with the purR ::ΦNΣ mutant met humane endpoint criteria by 24 hpi, whereas 100% of the mice infected with either the WT or complemented mutant survived past 72 hpi (Fig. 4a ). 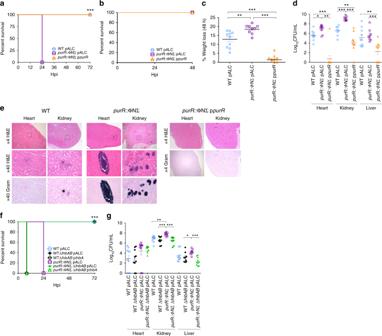Fig. 4 AS. aureus purRmutant is hypervirulent via FnbAB. Ina, mice (9–12 per group) were infected with ~1 × 107CFU of WT USA300, USA300purR::ΦNΣ or complementedpurR::ΦNΣ mutant and survival monitored over 72 h. ***p-value < 0.001, based on a Mantel-Cox test. Inb, animals were infected as ina, but with 2–2.5 × 106CFU, andcweight loss monitored daily for 48 h. **p-value < 0.01, ***p-value < 0.001, based on a one-way ANOVA with a Bonferroni post-test. Ind, animals frombwere sacrificed at 48 h post infection (hpi), and heart, kidney and liver were harvested and bacterial burdens determined. Data shown are mean ± SEM, *p-value < 0.05, **p-value < 0.01, ***p-value < 0.001, based on a Student’s unpairedt-test. Ine, two animals per bacterial strain were infected as ina, with ~1 × 107CFU, sacrificed at 24 hpi and organs harvested. Organs were paraffin embedded, sectioned and stained with H&E and a Gram stain. Representative images are shown. Inf, animals were infected as ina, with ~1 × 107CFU, with the inclusion of WTΔfnbABandpurR::ΦNΣΔfnbABstrains, and monitored for 72 h. ***p-value < 0.001, based on a Mantel-Cox test. Ing, the heart, kidney and liver from the animals infected inewere harvested at the point of sacrifice and bacterial burden determined. Data shown are mean ± SEM, *p-value < 0.05, **p-value < 0.01, ***p-value < 0.001, based on a Student’s unpairedt-test. Source data are provided as aSource Datafile The purR Q52P mutant demonstrated the same hypervirulent phenotype as the purR ::ΦNΣ mutant (Supplementary Figure 4a ). Fig. 4 A S. aureus purR mutant is hypervirulent via FnbAB. In a , mice (9–12 per group) were infected with ~1 × 10 7 CFU of WT USA300, USA300 purR ::ΦNΣ or complemented purR ::ΦNΣ mutant and survival monitored over 72 h. *** p -value < 0.001, based on a Mantel-Cox test. In b , animals were infected as in a , but with 2–2.5 × 10 6 CFU, and c weight loss monitored daily for 48 h. ** p -value < 0.01, *** p -value < 0.001, based on a one-way ANOVA with a Bonferroni post-test. In d , animals from b were sacrificed at 48 h post infection (hpi), and heart, kidney and liver were harvested and bacterial burdens determined. Data shown are mean ± SEM, * p -value < 0.05, ** p -value < 0.01, *** p -value < 0.001, based on a Student’s unpaired t -test. In e , two animals per bacterial strain were infected as in a , with ~1 × 10 7 CFU, sacrificed at 24 hpi and organs harvested. Organs were paraffin embedded, sectioned and stained with H&E and a Gram stain. Representative images are shown. In f , animals were infected as in a , with ~1 × 10 7 CFU, with the inclusion of WTΔ fnbAB and purR ::ΦNΣΔ fnbAB strains, and monitored for 72 h. *** p -value < 0.001, based on a Mantel-Cox test. In g , the heart, kidney and liver from the animals infected in e were harvested at the point of sacrifice and bacterial burden determined. Data shown are mean ± SEM, * p -value < 0.05, ** p -value < 0.01, *** p -value < 0.001, based on a Student’s unpaired t -test. Source data are provided as a Source Data file Full size image In subsequent experiments, we tested the effect of a lower dose of the purR ::ΦNΣ mutant and found that infection with ~2 × 10 6 CFU allowed survival up to 48 hpi (Fig. 4b ). At 48 hpi, we observed significantly greater weight loss and increased bacterial burdens in mice infected with the purR ::ΦNΣ mutant when compared to those infected with WT (Fig. 4c, d ). The mice infected with the complemented strain showed statistically significant decreases in weight loss and bacterial burden, even compared to mice infected with WT. Histopathological analysis of animals infected with a high dose of WT (~1 × 10 7 CFU) for 24 h demonstrated lesions predominantly in the heart and the kidney (Fig. 4e ). Animals infected with the purR ::ΦNΣ mutant had larger and more frequent lesions in both the heart and kidneys (Supplementary Table 2 ), with multifocal necrotic areas, often centred on discrete groups of Gram-positive bacteria (Fig. 4e ). Complementation of the purR ::ΦNΣ mutant almost completely eliminated the formation of lesions (Fig. 4e ), concurring with the decreased bacterial burden previously observed. To confirm the role of fnbAB in the purR hypervirulence phenotype, we infected mice with the Δ fnbAB mutant, in either the WT or purR ::ΦNΣ background. While purR ::ΦNΣ infected animals required sacrifice by 24 hpi the deletion of fnbAB in that background completely ablated the hypervirulent phenotype (Fig. 4f ). Of note, infections with strains carrying an fnbA overexpression plasmid, indifferent of the purR background, resulted in very rapid effects on animal health, and animals required euthanasia by ~6–8 hpi (Fig. 4f ). This demonstrates the profound effects of aberrant fnb overexpression, suggesting that even transient upregulation of FnBPs has a severe impact on disease severity in a systemic infection model. Bacterial burdens in the hearts, kidneys and livers of the remaining groups were in agreement with the survival data, with increased numbers of bacteria for the purR ::ΦNΣ strain, but not for the purR ::ΦNΣ Δ fnbAB strain, compared to WT (Fig. 4g ) (CFU for p fnbA carrying strains were not determined). Of note, no difference in survival or bacterial burden was observed between the WT and Δ fnbAB strains, indicating that while these proteins are not required for pathogenesis of WT USA300 in a systemic model of infection, they are indispensable for the hypervirulent phenotype of the purR ::ΦNΣ mutant. In agreement with the requirement of FnbAB for purR -dependent hypervirulence, a purR ::ΦNΣ mutant in strain Newman was not hypervirulent in this model (Supplementary Figure 4b ). Mutations in purR occur at elevated temperatures and in vivo The purR Q52P SNP and the purR V229frameshift SNP-containing strains were isolated following allelic replacement mutagenesis techniques, a process that has previously been reported to select for mutations in the virulence regulatory genes saeRS [16] . Plasmids for allelic replacement are often temperature sensitive and curing of plasmids following homologous recombination necessitates growth at elevated temperatures. To investigate if exposure to high temperatures also selects for purR mutations in S. aureus , we constructed a reporter strain that colorimetrically identifies purR mutants. 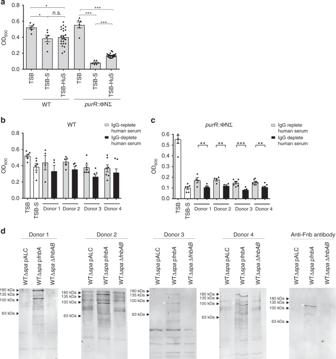Fig. 5 Anti-staphylococcal antibodies amelioratepurRhyper-clumping.aWT or thepurR::ΦNΣ mutant were grown in TSB, TSB-S or TSB with 10% v/v fresh human serum (TSB-HuS) for 3 h and relative clumping ability was measured using OD600as described above. Data shown are mean ± SEM of four independent experiments. *p-value < 0.05, **p-value < 0.01 and ***p-value < 0.001, based on a one-way ANOVA with a Bonferroni post-test. WT (b) or thepurR::ΦNΣ mutant (c) were grown in TSB (white bars), TSB-S (white bars), TSB-HuS (grey bars) or TSB with IgG-depleted human serum (HuS) (black bars) for 3 h and relative clumping ability measured as above. Data shown are mean ± SEM of four experiments, with four donors. **p-value < 0.01, ***p-value < 0.001, based on a one-way ANOVA with a Bonferroni post-test. Ind, whole cell lysates of WT, WT pfnbAor WTΔfnbABwere used for western blots, with human serum (from donors in panelsbandc) or a rabbit anti-Fnb serum (far right blot) used as a source of primary antibody. Source data are provided as aSource Datafile Given that the promoter of the purine biosynthetic operon ( purEKCSQLFMNHD ) was highly expressed in a purR mutant, we fused the promoter of this operon to a promoterless gusA gene, encoding ß-glucuronidase (referred to as P purE::gusA ) (Supplementary Figure 5a ), and inserted this fusion into the genome (see the Methods section). When cultured on X-Gluc-containing solid media, USA300 P purE::gusA colonies were pale yellow while the USA300 purR ::ΦNΣ strain carrying the genomic reporter were dark blue; this indicates that the reporter was capable of identifying purR mutants in culture. To define whether we could identify naturally-occurring purR mutants, we cultured USA300 P purE::gusA at either 37 °C or 42 °C, with daily passage, for 5 days. Blue colonies were only detected from cultures grown at 42 °C (Supplementary Figure 5b ), at a frequency of ~0.1–1.0% following 5 days of passaging (Supplementary Figure 5b ). Sequencing of the purR gene from select blue colonies identified a variety of additional mutations in purR (Y71Stop, V156E, S172Stop, H225D, S230Stop, Q240Stop). The in vivo environment also presents a strong selection pressure on bacteria. Therefore, we were interested to determine if passage of S. aureus through mice would select for purR mutants. Unfortunately, for unknown reasons, the USA300 P purE::gusA construct was lost from the genome without antibiotic selection in vivo. Therefore, we tested colonies recovered from the organs of mice infected with WT USA300 for 4 days for clumping in TSB-S (in a 96-well plate format). Potential mutants were phenotypically confirmed in a tube assay and the purR gene sequenced. A mutant with a R96A SNP was identified from an infected kidney, and demonstrated cell clustering in TSB (Supplementary Figure 5c ) and clumping in TSB-S (Supplementary Figure 5d ). The phenotype could be complemented by the introduction of p purR , indicating the SNP was solely responsible for the observed phenotype (Supplementary Figure 5c, d ). It was of interest whether strains containing SNPs in purR , and recovered from murine infections, also displayed the characteristic hypervirulence we described here. Infection of mice with the purR R96A SNP resulted in the same hypervirulent phenotype as the purR ::ΦNΣ mutant (Supplementary Figure 5e ), with animals requiring sacrifice within 24 hpi. Anti-FnBP antibodies ameliorate purR mutant clumping To date, despite the hypervirulence phenotype of purR mutation described above, no associations of purR mutations with human infection have been noted. A search of publicly available whole genome sequences identified a non-synonymous change or changes in the purR gene in 331 of 8201 sequences (Supplementary Data 1 ). However, few details on the infection type or outcome were available and, at this point, no correlations could be drawn between the presence of a purR mutation and disease severity. To begin to explore this further in the laboratory setting, we tested whether human serum can support hyper-clumping of purR ::ΦNΣ bacteria. We isolated fresh human serum from healthy volunteers and this serum was used to assay for clumping as described above. When the WT and purR ::ΦNΣ mutant were grown in TSB with 10% v/v human serum (TSB-HuS), the purR ::ΦNΣ clumped but clumping was less pronounced than that seen in horse serum (Fig. 5a ). Since the clumping phenotype relies on FnbA and FnbB, and their interaction with Fn, we hypothesised that anti-FnBP (i.e. blocking) antibodies are present in human serum, since humans are exposed to S. aureus throughout their lifetime, and that these antibodies would interfere with clumping. To test this, we passed human serum through a protein A column to remove IgG. TSB containing 10% v/v IgG-depleted human serum showed increased levels of clumping for the purR ::ΦNΣ mutant, when compared to TSB-HuS, but no significant difference was observed for the WT (Fig. 5b, c ). 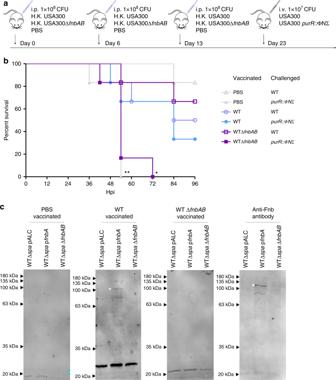Fig. 6 Vaccination withS. aureusexpressing FnbAB is protective against a challenge with apurRmutant.aVaccination scheme, with six animals per group.bSurvival of animals challenged with 1 × 107CFU of WT orpurR::ΦNΣS. aureusfollowing vaccination, as outlined ina. *p-value < 0.05, **p-value < 0.01, based on a Mantel-Cox test, as compared to WT vaccinated,purR::ΦNΣ challenged animals.cWhole cell lysate of WT, WT pfnbAor WTΔfnbABwere used for a western blot, with serum from vaccinated animals or a rabbit anti-Fnb serum (far right) used as a primary antibody Moreover, addition of the purified human IgG to the purR ::ΦNΣ mutant growing in TSB-S resulted in significant reduction of the clumping phenotype (Supplementary Figure 6 ). This indicates that antibodies present in human serum can interfere with the purR -dependent clumping phenotype. Western blot analysis determined that human serum did indeed contain anti-FnbA/B antibodies (Fig. 5d ); while no signal could be detected for the WT, likely due to low expression, which is in agreement with our luminescence findings (Fig. 3c ), bands could be visualised if a strain carried an fnbA overexpression construct. These data indicate that humans carry anti-FnbA/B antibodies that, while not necessarily protective against S. aureus infection, may confer protection against the hyper-virulent purR phenotype. Fig. 5 Anti-staphylococcal antibodies ameliorate purR hyper-clumping. a WT or the purR ::ΦNΣ mutant were grown in TSB, TSB-S or TSB with 10% v/v fresh human serum (TSB-HuS) for 3 h and relative clumping ability was measured using OD 600 as described above. Data shown are mean ± SEM of four independent experiments. * p -value < 0.05, ** p -value < 0.01 and *** p -value < 0.001, based on a one-way ANOVA with a Bonferroni post-test. WT ( b ) or the purR ::ΦNΣ mutant ( c ) were grown in TSB (white bars), TSB-S (white bars), TSB-HuS (grey bars) or TSB with IgG-depleted human serum (HuS) (black bars) for 3 h and relative clumping ability measured as above. Data shown are mean ± SEM of four experiments, with four donors. ** p -value < 0.01, *** p -value < 0.001, based on a one-way ANOVA with a Bonferroni post-test. In d , whole cell lysates of WT, WT p fnbA or WTΔ fnbAB were used for western blots, with human serum (from donors in panels b and c ) or a rabbit anti-Fnb serum (far right blot) used as a source of primary antibody. Source data are provided as a Source Data file Full size image Anti-FnBP antibodies protect against purR hypervirulence Given our data indicated that anti-FnbA/B antibodies present in human serum can impair purR mutant clumping, we hypothesised that mice with antibodies recognizing the FnBPs would be protected from hypervirulence associated with purR ::ΦNΣ infection. To test this, we vaccinated groups of 12 mice intraperitoneally with either 1 × 10 8 heat-killed (HK) USA300, 1 × 10 8 HK USA300Δ fnbAB , or with PBS on day 0, 6 and 13 (Fig. 6a ). On day 23, animals in each group were challenged with either live WT USA300 or USA300 purR ::ΦNΣ bacteria. In groups vaccinated with WT USA300, significantly more animals survived challenge with the purR ::ΦNΣ strain, when compared to those vaccinated with USA300Δ fnbAB or the vehicle control (Fig. 6b ). Serum from vaccinated animals demonstrated that mice receiving HK WT USA300 raised antibodies towards S. aureus antigens, including FnbA/B, while those challenged with HK USA300Δ fnbAB likewise raised antibodies to many antigens, but not to FnbA/B proteins (Fig. 6c ), indicating the protective response is indeed due to anti-FnbA/B antibodies. Fig. 6 Vaccination with S. aureus expressing FnbAB is protective against a challenge with a purR mutant. a Vaccination scheme, with six animals per group. b Survival of animals challenged with 1 × 10 7 CFU of WT or purR ::ΦNΣ S. aureus following vaccination, as outlined in a . * p -value < 0.05, ** p -value < 0.01, based on a Mantel-Cox test, as compared to WT vaccinated, purR ::ΦNΣ challenged animals. c Whole cell lysate of WT, WT p fnbA or WTΔ fnbAB were used for a western blot, with serum from vaccinated animals or a rabbit anti-Fnb serum (far right) used as a primary antibody Full size image Staphylococcus aureus is a prolific pathogen of humans and animals and, with the emergence of multi-drug resistant strains, efforts to uncover novel drug targets and deliverables have intensified. The discovery and characterisation of novel drug targets often necessitates genetic manipulation of the pathogen under investigation, yet during commonly employed mutagenesis procedures off-target mutations can be induced that profoundly influence the pathogenic potential of this bacterium. Here, we found that exposure of S. aureus to stress such as elevated temperatures (i.e. 42 °C during mutagenesis) or an active host immune response can induce loss of function mutations in the purR gene. PurR is a predicted transcriptional regulator of the purine biosynthetic operon as in other bacteria [28] , [29] , and expression of the pur operon is elevated in S. aureus purR mutants. The observation that exposure to stress induces purR mutations could suggest that increased purine biosynthesis is of benefit to S. aureus under these conditions. In E. coli exposure to elevated pH (i.e. pH ≥ 9.0) is also reported to induce purR mutations consistent with the notion that de-repression of the pur operon may promote bacterial survival during exposure to certain stresses [30] . Remarkably, inactivation of purR in S. aureus causes robust bacterial clumping in the presence of the extracellular matrix protein fibronectin, and causes hyper-virulence in a murine model of systemic infection. Interest in purine metabolism in S. aureus has emerged because disruption of purine biosynthetic pathways can yield growth defects and diminish virulence [31] , [32] , [33] , however, the contribution of the PurR regulator to the physiology of S. aureus has not, to our knowledge, been explored. Consistent with reports of reduced S. aureus fitness when purine biosynthesis is disrupted, we find that provision of PurR in trans reverses the enhanced virulence of purR ::ΦNΣ S. aureus USA300 and attenuates infection (see Fig. 5a ). Presumably, overexpression of PurR represses the purEKCSQLFMNHD biosynthetic operon, thereby mimicking the effects of a pur gene deletion, which renders S. aureus less able to grow in human blood and during infection [34] , [35] , [36] . How purine metabolism impacts S. aureus is unclear, but one possibility is that it involves the bacterial stringent response, which could conceivably enhance resistance to stress. In S. aureus the stringent response can be induced upon amino acid starvation and exposure to the antibiotic mupirocin [37] , and to the cell wall-targeting antibiotic vancomycin [38] . Interestingly, exposure to mupirocin and activation of the stringent response has been shown to repress expression of multiple Pur proteins such as PurE, PurQ, and PurK and have a more global impact on gene expression [39] . Contrary to these findings, our RNAseq data revealed that purR ::ΦNΣ S. aureus demonstrated upregulation of pur genes, but no global changes in gene expression, arguing that deletion of the purR gene in S. aureus is unlikely to evoke the stringent response. The hypervirulent phenotype of purR ::ΦNΣ S. aureus is dependent on expression of fibronectin binding proteins A and/or B (FnbA/B) and deletion of the tandemly-duplicated fnbAB genes ablates lethality of the purR ::ΦNΣ mutant. FnbA/B are known to bind the extracellular matrix proteins fibronectin and fibrinogen, and contribute to the adhesion of wild-type S. aureus to host tissues, to mediate cellular invasion, and promote virulence during infection [40] , [41] , [42] . Our analysis of fnbA and fnbB gene expression reveals that PurR plays a heretofore undescribed role in repressing FnbA/B expression. Our data support the notion that PurR negatively regulates FnBP expression in early log-phase cells and de-repression of FnBP transcription in purR deficient bacteria occurs only transiently, indicating additional regulatory factors also coordinate FnBP expression. Indeed, previous work characterizing FnbA expression has demonstrated that the global regulators of staphylococcal virulence Agr and Sar coordinate FnbA expression [43] , [44] . Nevertheless, aberrant regulation of FnbA/B expression in S. aureus purR mutants plays a vital role in the hyper-agglutination and the hypervirulent phenotypes described herein. Furthermore, the importance of carefully regulated FnBP expression during S. aureus infection is also evidenced by experiments where constitutive expression of plasmid encoded fnbA causes lethal S. aureus infection irrespective of purR (Fig. 4f ). At present it is unclear what mechanism within the host causes mortality. However, due to the fact that FnBP proteins promote bacterial clumping and/or interaction with host platelets [45] , [46] , it is tempting to speculate that thrombus formation may be a contributing factor. Our data also reveal that FnbA/B contribute significantly to colonization of kidney and liver tissue by purR ::ΦNΣ S. aureus during systemic infection. This contrasts wild-type USA300 where FnbA/B expression seems to play a less important role, as deletion of the fnbA/B genes alone did not significantly affect colonization of the murine heart, kidney or liver (see Fig. 4g ). Presumably this can be attributed, in part, to the multitude of virulence factors that S. aureus can express and their potential redundancy. The relative differences in the contribution of FnBP proteins to the pathogenesis of wild-type S. aureus USA300 and in the purR ::ΦNΣ strain is also evident from our vaccination study, where immunization of mice with FnbA/B-expressing S. aureus conferred protection against purR ::ΦNΣ lethality but was largely without effect on wild-type USA300 infection. The differences observed in purR ::ΦNΣ bacterial clumping in human versus horse serum prompted our consideration for the existence of anti-staphylococcal antibodies directed to the FnBPs of S. aureus , as has previously been reported [47] , [48] . Human sera do contain naturally occurring anti-FnbA/B antibodies and the presence of these antibodies correlates with reduced purR bacterial clumping in human serum (see Fig. 5 ). Importantly, these data suggest that some of these naturally occurring antibodies neutralize FnBP-Fn interactions, and the presence of these immunoglobulins may confer protection against the potentially severe consequences of infection with S. aureus purR variants that may arise in humans. Several attempts have been made to create an anti- S. aureus vaccine however, to date, no vaccine has successfully protected against human infection [49] , [50] , [51] , [52] . Despite this, it is conceivable that immunization with certain S. aureus antigens may offer protection against aspects of staphylococcal pathogenesis (e.g. FnbA/B-dependent events) without altogether preventing infection, a notion that is supported by our data. Nevertheless, the pursuit of a vaccine that will protect against S. aureus infection over and above naturally occurring humoral immunity represents an important aim that will likely require a better understanding of human infection by S. aureus . In summary, we have discovered that mutations in the S. aureus purR gene, arising from exposure of S. aureus to routine genetic manipulation or to the murine infection environment, can profoundly impact the pathogenesis of this bacterium. Hypervirulence associated with strains carrying purR mutations would undoubtedly offset the potentially desired attenuation phenotype associated with the mutation under study, severely confounding the interpretation of results of S. aureus virulence studies. As such, we urge S. aureus investigators to judiciously characterize mutant strains for off-target mutations affecting toxin production (e.g. sae , as previously reported) and purR , the latter easily tested by growing strains in media containing horse serum. The use of next generation sequencing makes identifying these and other off-target mutations straight forward. Our data show that the mechanism of purR mutant hypervirulence occurs via increased expression of fibronectin binding proteins at low cell densities. The detailed in vivo events occurring during infection of mice with S. aureus purR mutants are currently under study in our laboratory. Bacterial growth conditions Bacterial strains and plasmids used in this study are listed in Table 1 and primers are listed in Table 2 . E. coli was grown in Luria-Bertani (LB) broth and S. aureus was grown in tryptic soy broth (TSB) at 37 °C, shaken at 200 rpm, unless otherwise stated. Where appropriate, media were supplemented with erythromycin (3 µg/mL), chloramphenicol (12 µg/mL), lincomycin (10 µg/mL), ampicillin (100 µg/mL) or tetracycline (3 µg/mL). Solid media were supplemented with 1.5% (w/v) Bacto agar. Table 1 Bacterial strains used in this study Full size table Table 2 Primers used in this study Full size table PCR and construct generation S. aureus strain USA300 LAC, cured of the 27-kb plasmid that confers antibiotic resistance, was used as the WT strain for mutant generation, unless otherwise stated. For mobilizing transposon insertion mutations into various genetic backgrounds, phage transduction was performed according to standard techniques. Phage lysate was prepared from the donor strain using phage 80α, recipient strains were infected and transductants selected using appropriate antibiotics. Insertions were confirmed by PCR. Markerless deletions were constructed using the pKOR1 system, as previously described [53] . Briefly, upstream and downstream regions flanking the FnbAB genes were amplified with primers FnbAB Up F and Up R, and FnbAB Down F and Down R, respectively, using Phusion DNA polymerase and recombined into pKOR1. The resulting vector was passaged through RN4220 and subsequently introduced into strains of interest by electroporation. Genomic deletions were confirmed by PCR with primers hybridizing outside of the cloned area of interest. The purE promoter-glucuronidase fusion reporter was synthesised by Integrated DNA Technologies (IDT, Canada), and ligated into pLL29. pLL29 was transformed into RN4220 containing a plasmid encoding an integrase and later transduced into USA300 and derivatives [54] . For complementation with WT purR or fnbA , the full-length genes were amplified using primers PurR F and PurR R and FnbA F and FnbA R, respectively, ligated into pALC2073 and recombinant plasmids transformed into E. coli . Plasmids were then passaged through RN4220, prior to transformation into the strain of interest. For insertion of fnb promoters into pGYlux, sequences were amplified from the USA300 genome with primer pairs pGYluxFnbA F and pGYluxFnbA R (for pGY: fnbA) and pGYluxFnbB F and pGYluxFnbB R (for pGY:: fnbB) , respectively. Constructs were passaged through RN4220, prior to transformation into the strain of interest. Clumping assays For measurement of clumping in serum (horse or human), overnight cultures in TSB were diluted to OD 600 0.03 in 2 mL TSB or TSB with 10% (v/v) serum in a 13 mL tube and grown at 37 °C, with shaking at 200 rpm for 3.5 h. Cultures were allowed to sit without shaking for 5 min and the OD 600 of the middle of the culture was determined. The same cultures were imaged live on a brightfield Leica microscope at ×40 magnification. Fibronectin removal To remove fibronectin from horse serum, sterile, heat-inactivated horse serum was passaged over a column of gelatin sepharose (GE healthcare) (column bed volume of 5.5 mL) at ~1 mL/min and the flow through collected. The column was washed with ~20 mL of phosphate-buffered saline (PBS) and bound fibronectin was eluted with PBS + 4 M urea. The column was re-generated as per manufacturer’s instructions and the run-through from the first purification passaged again. A total of three passages over the column were performed and the fibronectin-free serum was sterilized by passage through a 0.22 µm filter. The different run troughs were used at 10% (v/v) in standard clumping assays, as described above. Electron microscopy S. aureus strains were grown in TSB or TSB with 10% horse serum for 3.5 h, as previously described for clumping assays. The bacteria were then fixed overnight with a modified Karnovsky’s fixative (2.5% glutaraldehyde (v/v) + 2% paraformaldehyde (v/v) in 0.1 M cacodylate buffer, pH 7.2). The fixed bacteria were embedded in a 1% (w/v) agarose suspension and post-fixed with 1% (w/v) osmium tetroxide for 2 h, followed by a 2-h en bloc 0.5% (w/v) uranyl acetate strain. Samples were then progressively dehydrated with 15-min treatments of increasingly concentrated ethanol solutions (50, 70, 90, 95, 100% (v/v)). After dehydration, the samples were embedded in Epon-Araldite and ultrathin sections (70 nm) were cut and placed on nickel grids using an Ultracut microtome. The cut samples were surface stained for 15 min with 0.5% (w/v) uranyl acetate and viewed with a Phillips 420 transmission electron microscope equipped with a Hamamatsu Orca 2 MPx HRL camera. Preparation of proteins For examination of secreted protein profiles, strains were grown to the desired OD 600 in TSB and normalised to OD 600 of 6.0, pelleted by centrifugation, and supernatant mixed with 100% ethanol at a 1:3 ratio. Samples were incubated at −20 °C for 4–8 h and proteins pelleted at 5000 × g for 30 min at 4 °C. Pellets were re-suspended in 1:20th of the original cultured volume in PBS and stored at −20 °C. For whole cell lysate preparation, cells grown to the desired density were pelleted, washed once with PBS, re-suspended in 1:20th of the original volume in PBS with 400 µg lysostaphin and incubated at 37 °C for 1 h. Samples were passaged twice through a Cell-Disruptor (Constant Systems Ltd.) at 34,000 p.s.i., pelleted at 5000 × g for 10 min and supernatant harvested. For mass spectrometry analysis of bacterial clumps, the purR::ΦΝΣ mutant strain was grown in TSB with 10% (v/v) for 3 h at 37 °C, and clumps allowed to settle at the bottom of the tube. Clumps were washed three times with PBS, dissolved in 1% SDS at 55 °C for 1 h and run on a 7% SDS polyacrylamide gel. Bands of interest were picked for LC-MS-MS analysis. Western blots Strains used for Western blot analysis were the same as described above, with the additional deletion of protein A ( spa) and sbi , to eliminate non-specific IgG interactions. Whole cell lysate was prepared as described above, mixed with 1× Laemmli buffer (60 mM Tris-HCl, pH 6.8, 2% (w/v) SDS, 10% (v/v) glycerol, 5% (v/v) β-mercaptoethanol, 0.01% (w/v) bromphenol blue), boiled for 10 min and separated on a 10% polyacrylamide gel. Following electrophoresis, proteins were transferred to a nitrocellulose membrane following standard protocols. Human, mouse or horse sera (1:500 dilution) or rabbit anti-FnbA antiserum [55] (1:500 dilution) were used as a primary antibody, and secondary antibody (conjugated to IRDye 800; Li-Cor Biosciences, Lincoln, NE) was used at a 1:20,000 dilution. Membranes were scanned on a Li-Cor Odyssey Infrared Imager (Li-Cor Biosciences) and visualized using Odyssey Version 3.0 software. Biofilm assay Biofilm assays were performed as described previously [56] . Briefly, 200 µL of TSB supplemented with 0.4% w/v glucose was inoculated with a 1:100 dilution of an overnight culture. After static incubation at 37 °C for 16–22 h, cells were washed three times with PBS and fixed by drying at 42 °C. Crystal violet (0.4% (w/v)) was used to stain cells for 15 min, before being dissolved in glacial acetic acid (10% (v/v)) and level of adhesion quantified by absorbance at 595 nm. Absorbance was normalized to the WT strain, which was set to 1. Luciferase-based measurements of fnb promoter activity WT or purR ::ΦNΣ strains carrying pGYlux constructs with the promoter of fnbA (pGY:: fnbA ) or fnbB (pGY:: fnbB ) were used. For luciferase measurements, overnight cultures grown in TSB with chloramphenicol were diluted to OD 600 of 0.01 in TSB with chloramphenicol and 200 µl added to a white optical 96-well plate (Thermo Fisher). Growth and luminescence were measured in a BioTek Synergy H4 plate reader at 37 °C with shaking. Data for both absorbance and luminescence was normalised to blank measurements for each time point. RNA extraction and RNAseq S. aureus strains were grown overnight, subcultured to an OD 600 equivalent of 0.01 in TSB and grown to the desired growth phase. Cells equating to an OD 600 of 3.0 were harvested for each culture, and RNA extraction was performed by E.Z.N.A® total RNA kit (Bio-Rad) according to the manufacturer’s instructions with the addition of 0.25 μg/mL lysostaphin to the lysis solution. RNA purity was determined by visualisation on an agarose gel, and RNA concentration was determined by NanoDrop® ND-1000 UV-Vis spectrophotometer. cDNA preparation was performed using 500 ng of total cellular RNA reverse-transcribed using Superscript TM II reverse transcriptase (Invitrogen) according to the manufacturer’s instructions. For each qPCR, 1 μg of cDNA was amplified in a Rotor-Gene 6000 (Corbett Life Science) using the iScript One-Step RT-PCR kit with SYBR Green (Bio-Rad). Gene expression for each sample was quantified in relation to rpoB expression. A standard curve was generated for each gene examined. For RNAseq, RNA was extracted as above, a library was constructed using an Illumina Script Seq RNA sequencing kit and sequenced on an Illumina MiSeq. Genome sequence analysis The nucleotide sequence of the purR gene was downloaded from 8207 S. aureus available genome sequences or assemblies from the NCBI database (1st Dec 2017). Sequences were translated and amino acids aligned to the USA300 LAC purR sequence using MEGA 7. For strains with sequence changes as compared to USA300 FPR3757, the information available was compiled into Supplementary Data 1 . Ethics statements Human blood was obtained from healthy adult volunteers, with written permission and in compliance with protocol 109059 approved by the Office of Research Ethics at the University of Western Ontario. All animal experiments were performed in compliance with guidelines set out by the Canadian Council on Animal Care. All animal protocols (protocol 2017-028) were reviewed and approved by the University of Western Ontario Animal Use Subcommittee, a subcommittee of the University Council on Animal Care. Human serum antibody removal Blood was allowed to clot for 30 min at RT, centrifuged at 400 × g for 10 min (no brake) and serum harvested. Serum was filtered through a 0.22 µm filter and heat-inactivated for 1 h at 56 °C. For removal of antibody, 4 mL serum was loaded on a HiTrap protein A column (GE healthcare) at 1 mL/min, followed by a 15 min wash (20 mM sodium phosphate, pH 7) at 1 mL/min. Antibody was eluted (0.1 M sodium citrate, pH 4) in three fractions (1.5 mL/each) at 1 mL/min. Serum used for clumping assays was passaged through the column twice. Eluted IgG was filtered through a 0.22 µm filter, concentrated with an Amicon ultra-50 centrifugal filter and added to clumping assays containing 10% (v/v) horse serum. Mouse infections Six- to eight-week-old female BALB/c mice (Charles River laboratories) were injected via tail vein with 100 µL of bacterial culture, containing 1 × 10 6 –1 × 10 7 CFU of bacteria, as described in the text. To prepare the bacteria, strains were grown to OD 600 2–2.5 in TSB, washed twice with PBS and re-suspended to the desired OD 600 in PBS. Infections were allowed to proceed for up to 96 h before animals were euthanized, or when they met guidelines for early euthanasia. Organs were harvested in PBS + 0.1% Triton X-100 (Sigma), homogenised in a Bullet Blender Storm (Next Advance, Troy, NY), using two runs of 5 min at setting 10, and metal beads. Dilutions of organ homogenates were plated on TSA for CFU enumeration. For vaccination studies, bacteria were grown to OD 600 of ~0.6, bacteria washed as above, heat killed at 85 °C for 15 min and 100 µL, equivalent to ~1 × 10 8 CFU, were injected intraperitoneally (IP). For challenge post vaccination, infections were as outlined above. Statistical analysis Statistical analyses were performed with GraphPad Prism software v5.0 or v7.0. Reporting Summary Further information on experimental design is available in the Nature Research Reporting Summary linked to this Article.